Ribosome profiling reveals features of normal and disease-associated mitochondrial translation Mitochondria are essential cellular organelles for generation of energy and their dysfunction may cause diabetes, Parkinson’s disease and multi-systemic failure marked by failure to thrive, gastrointestinal problems, lactic acidosis and early lethality. Disease-associated mitochondrial mutations often affect components of the mitochondrial translation machinery. Here we perform ribosome profiling to measure mitochondrial translation at nucleotide resolution. Using a protocol optimized for the retrieval of mitochondrial ribosome protected fragments (RPFs) we show that the size distribution of wild-type mitochondrial RPFs follows a bimodal distribution peaking at 27 and 33 nucleotides, which is distinct from the 30-nucleotide peak of nuclear RPFs. Their cross-correlation suggests generation of mitochondrial RPFs during ribosome progression. In contrast, RPFs from patient-derived mitochondria mutated in tRNA-Tryptophan are centered on tryptophan codons and reduced downstream, indicating ribosome stalling. Intriguingly, long RPFs are enriched in mutated mitochondria, suggesting they characterize stalled ribosomes. Our findings provide the first model for translation in wild-type and disease-triggering mitochondria. The primary function of the mitochondrion is ATP production via the oxidative phosphorylation pathway [1] . The human mitochondrial genome contains 37 genes of which 13 are protein-coding. These genes are essential for normal energy production function of the mitochondria but also other processes such as cell signaling and cell death [2] , [3] . The mitochondria harbor their own ribosomes, which are structurally more similar to bacterial ribosomes than the cytosolic ribosomes [4] . However, the protein-synthesizing system of mitochondria and the template mRNAs contain unique features not observed in prokaryotes or the eukaryotic cell cytosol, including arginine codons AGG and AGA, which are unassigned while UGA stop codon codes for tryptophan; both AUG and AUA serve as START codons; messenger RNAs (mRNAs) essentially lack untranslated regions, are uncapped and contain a poly(A) tail, and mitochondria use a simplified decoding mechanism that allows translation of all codons with only 22 tRNAs [1] . Because of their function in the oxidative phosphorylation pathway, mitochondria are recognized for their role in the production of reactive oxygen species (ROS) and nitric oxide [5] . The production of ROS may also be associated with ageing since mitochondria increase production of ROS during human lifespan [6] . Interestingly, mutations in mitochondrial translation machinery, such as their tRNAs, are the source of various human diseases, typically causing multi-systemic disorders and early fatality [7] . To characterize mitochondrial translation we used ribosome profiling, a deep sequencing-based technology that allows quantitative analysis of translation at nucleotide resolution [8] , [9] . Ribosome profiling maps the positions of ribosomes on transcripts by nuclease footprinting, generating nuclease-protected mRNA fragments bound to ribosomes that are converted into a DNA library suitable for deep sequencing. We observed a poor capacity of the established ribosome profiling protocol to capture mitochondrial ribosome protected fragments (RPFs) and developed a suitable method for this purpose. We then used the adapted protocol to show that the mitochondrial tRNA(Trp) 5556G>A mutation induces strong ribosome stalling. Mitochondrial RPFs are poorly captured by current protocols The abundance of RPFs was demonstrated to correlate with the level of translation of a gene [8] . 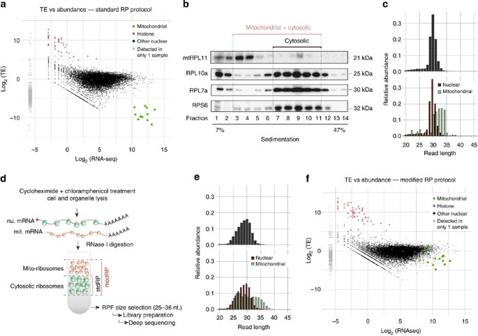Figure 1: A modified ribosomal profiling protocol improves detection of mitochondrial translation. (a) A plot showing the TE as a function of mRNA abundance in a standard ribosomal profiling protocol. Mitochondrial and histone genes (in green and red, respectively) appear as outside groups. (b) Western blot showing the abundance of mitochondrial (mtRPL11) and cytosolic (RPL10a, RPL7 and RPS6) ribosomal proteins in different sucrose gradient fractions after RNAse I treatment. (c) Size distribution of RPFs in the standard ribosome profiling. The upper panel shows all reads, the lower panel shows nuclear-encoded genes (red) and mitochondrially encoded genes (green) separately. (d) Overview of our modified ribosome profiling protocol. (e) Size distribution of RPFs obtained by our modified ribosome profiling. (f) Same as inafor modified protocol. Marked improvement in the detection of TE in mitochondrial genes is observed. Figure 1a shows the translational efficiency (TE; normalized abundance measured by ribosome profiling divided by normalized abundance measured by RNA sequencing) of nuclear- and mitochondrial-encoded genes. Curiously, all mitochondrial transcripts (marked green) showed a high level of signal in the RNA-seq while having a very low amount of reads in the ribosome profiling data compared with the bulk of the nuclear transcripts, which had TE values centered on the norm and up to fourfold difference in the vast majority of the cases, resulting in relatively low TE values for mitochondrial genes. A similar observation was seen when we used several recently published ribosome profiling data sets [10] , [11] (see Supplementary Fig. S1 and Supplementary Table S1 ). In contrast, histone genes, which are not polyadenylated and therefore are poorly retrieved during mRNA sequencing, showed as expected relatively extremely high, TE values (marked red in Fig. 1a ). Figure 1: A modified ribosomal profiling protocol improves detection of mitochondrial translation. ( a ) A plot showing the TE as a function of mRNA abundance in a standard ribosomal profiling protocol. Mitochondrial and histone genes (in green and red, respectively) appear as outside groups. ( b ) Western blot showing the abundance of mitochondrial (mtRPL11) and cytosolic (RPL10a, RPL7 and RPS6) ribosomal proteins in different sucrose gradient fractions after RNAse I treatment. ( c ) Size distribution of RPFs in the standard ribosome profiling. The upper panel shows all reads, the lower panel shows nuclear-encoded genes (red) and mitochondrially encoded genes (green) separately. ( d ) Overview of our modified ribosome profiling protocol. ( e ) Size distribution of RPFs obtained by our modified ribosome profiling. ( f ) Same as in a for modified protocol. Marked improvement in the detection of TE in mitochondrial genes is observed. Full size image Two potential explanations can clarify the low detection level of mitochondrial genes in the ribosome profiling data. First, mitochondrial genes might be translated at a remarkably different rate compared with the cytosolic mRNAs. Alternatively, the ribosome profiling protocol does not efficiently capture mitochondrial RPFs as a result of either a distinct size of the mitochondrial ribosomes or a distinct size of RPFs protected by the mitochondrial ribosomes, compared to the nuclear-ribosomes. As mitochondrial ribosomes are very different from the nuclear ones, and mitochondrial proteins are produced in high rate, inefficient capturing of mitochondrial RPFs the RP protocol seems more likely. Therefore, we first determined the fractions where mitochondrial monosomes localize after RNAse I treatment and sucrose gradient sedimentation, and indeed this analysis indicated altered sedimentation ( Fig. 1b ). Second, we also examined the size of RPFs in mitochondrial- and nuclear-encoded genes. Figure 1c shows that while nuclear genes feature the expected enrichment of 30-nt long RPFs, the size distribution of mitochondrial RPFs is clearly larger and seems truncated. As the ribosome profiling protocol we used included a selection step for fragments sized 27–33 nt, this result suggests that most of the mitochondrial RPFs may have a different size and thus are vastly excluded during this selection step. Improving retrieval of mitochondrial RPFs We modified the ribosome profiling protocol to collect more mitochondrial ribosomes in the sucrose gradient and relaxed the size of RPFs cutoff to 25–36 during size excision of adapter ligated reads ( Fig. 1d ). Indeed, Fig. 1e demonstrates that this protocol results in RPFs whose global size distribution coincides with the expected expansion in fragments cutoff. Moreover, it also shows that while nuclear RPFs showed the expected peak at 30 nt, a much broader distribution of the mitochondrial RPFs with a bimodal size peaking at 27 and 33 nt was observed. Last, Fig. 1f shows that our modified ribosome profiling protocol indeed improved the apparent TE of mitochondrial mRNAs to levels comparable to the nuclear-encoded mRNAs without compromising the quality of libraries. As shown in Fig. 2a , the reproducibility between RP samples is high (R2 0.91), comparable to RNA-seq data ( Fig. 2b ). The data shows periodicity ( Fig. 2c ) and the modifications in the protocol do not lead to increase of ribosomal RNA contamination ( Fig. 2d ). Lastly, as a characteristic of ribosome profiling data, the vast majority of reads originate from CDSs and a steep increase in RPF density is observed at the START codons, and similarly, a steep decrease is observed at the STOP codons ( Fig. 2e ). 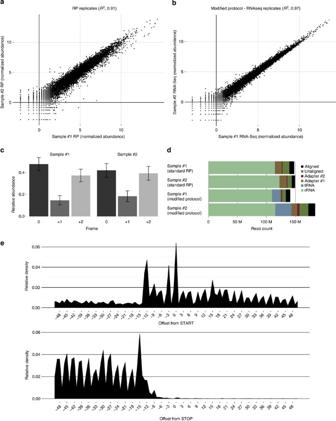Figure 2: Reproducibility and quality control of modified ribosome profiling protocol. (a) Correlation between ribosome profiling data set replicates in the modified ribosome profiling protocol. (b) Correlation between RNAseq data sets in the modified ribosome profiling samples. (c) In-frame RPF abundance for nuclear-encoded genes in two modified ribosome profiling replicate samples. Error bars indicate standard deviations across the genes with at least 100 RPFs (n=5579 for sample #1 andn=7108 for sample #2). (d) Abundances of mRNA and contamination in the conventional and modified ribosome profiling protocol samples. (e) Coverage around START and STOP codons in modified ribosome profiling sample #1. Figure 2: Reproducibility and quality control of modified ribosome profiling protocol. ( a ) Correlation between ribosome profiling data set replicates in the modified ribosome profiling protocol. ( b ) Correlation between RNAseq data sets in the modified ribosome profiling samples. ( c ) In-frame RPF abundance for nuclear-encoded genes in two modified ribosome profiling replicate samples. Error bars indicate standard deviations across the genes with at least 100 RPFs ( n =5579 for sample #1 and n =7108 for sample #2). ( d ) Abundances of mRNA and contamination in the conventional and modified ribosome profiling protocol samples. ( e ) Coverage around START and STOP codons in modified ribosome profiling sample #1. Full size image Mitochondrial RPF length shows bimodality The apparent bimodal distribution of mitochondrial RPFs length, peaking at 27 and 33 nt, may indicate alternative mitochondrial ribosome configurations or different positioning on mRNA. To examine this point we divided the mitochondrial RPFs into short (24–29 nt) and long (31–36 nt) fragments and measured their distribution over the mitochondrial transcripts. 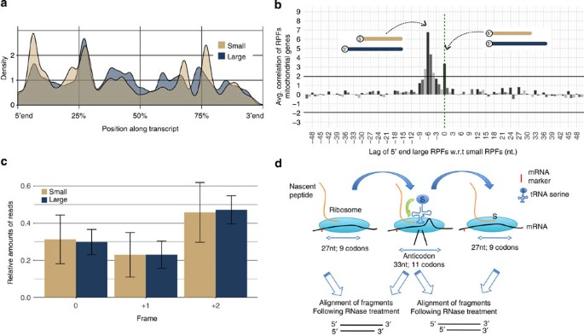Figure 3: Size distribution of mitochondrial RPFs suggests mechanism of action. (a) The normalized abundance of short and long RPFs along the 13 protein-coding mitochondrial genes. (b) Correlation between the 27 nt length (short) and 33 nt length (long) mitochondrial RPFs averaged over all mitochondrial protein-coding genes (n=13) in the control sample #1. Error bars indicate s.d.’s. (c) Normalized frame abundance of short and long RPFs on all mitochondrial protein coding genes. Error bars indicate s.d. across the mitochondrial protein-coding genes. (d) A schematic model showing how the long and short fragments might be produced during mitochondrial ribosome procession. Figure 3a shows an overall similar pattern of distribution between the two types of mitochondrial-RPFs, both were distributed similarly along the transcripts, though some positions were reproducibly slightly more enriched with one type of fragment. Additionally, analyzing the orientation of mitochondrial-RPFs with respect to the START codon, we found no apparent periodicity difference between the short and long fragments ( Fig. 3b ). These results may indicate that the two mitochondrial-RPF types are either generated from the same ribosome during the translation process, or from two types of related ribosomes both engaged in active translation of the mitochondrial genes. Interestingly, if the first is the case, a global correlation between the positions of the two types of RPFs should exist. We therefore compared the correlation between the distribution of reads with exactly 27 and 33 nt in length and found two preferential relationships ( Fig. 3c ). The peak at –6 indicates an overhang of 6 nt at the 5′ end, while the peak at 0 indicates alignment of the 5′ ends and thus an overhang of 6 nt at the 3′ end. Though not entirely excluding the existence of two separate mitochondrial ribosome types, this result strongly supports the hypothesis that the two RPF types are generated from one mitochondrial ribosome during its progression in a manner depicted in Fig. 3d . We envision that during progression the mitochondrial ribosome encompasses additional 6 nt. Figure 3: Size distribution of mitochondrial RPFs suggests mechanism of action. ( a ) The normalized abundance of short and long RPFs along the 13 protein-coding mitochondrial genes. ( b ) Correlation between the 27 nt length (short) and 33 nt length (long) mitochondrial RPFs averaged over all mitochondrial protein-coding genes ( n =13) in the control sample #1. Error bars indicate s.d.’s. ( c ) Normalized frame abundance of short and long RPFs on all mitochondrial protein coding genes. Error bars indicate s.d. across the mitochondrial protein-coding genes. ( d ) A schematic model showing how the long and short fragments might be produced during mitochondrial ribosome procession. Full size image tRNA(Trp) 5556G>A mutation causes ribosome stalling Next, to learn more about the protein translation process in mitochondria and relate it to mitochondria malfunction, we utilized trans-mitochondrial cybrids, rho(0) cells that lack mitochondrial DNA and fused with patient-derived mitochondria [12] . We performed our ribosomal profiling on cybrids containing either wild-type (wt) or the naturally occurring pathogenic mutant mitochondria at tRNA(Trp) 5556G>A , as this was shown to cause impairment of mitochondria function and reduce mitochondrial protein translation [12] . Although mitochondria-targeted TagYFP expression showed no major abnormalities in terms of number of mitochondria between wt and mutant mitochondria ( Supplementary Fig. S2A ), mitochondrial activity assays ( Table 1 ) and acidification of medium ( Supplementary Fig. S2B ) indicated reduced functionality, consistent with reported OXPHOS defects [12] . The mutation was verified using tRNA sequences retrieved in the ribosome profiling and purity was >99% ( Supplementary Fig. S5 ). Table 1 Enzymatic activity of respiratory complexes I–V in the tRNA(Trp) 5556G>A mutant cybrid and control cells. Full size table Intriguingly and most importantly, our ribosomal profiling method revealed a distinct distribution pattern of mitochondrial RPFs between wt and tRNA(Trp) 5556G>A mitochondria ( Fig. 4a ). In particular, peaks of the tRNA(Trp) 5556G>A mitochonderia typically tended to be centered on tryptophan codons. Data analysis confirmed increased abundance of RPFs with the mitochondrial-tryptophan codons TGA and TGG ( Fig. 4b ). Moreover, RPF alignment analysis indicated that the tryptophan codons are centered in the middle of the RPFs, positions 15–18, implying stalling of the ribosome when encountering tryptophan codons. This effect was specific to mitochondrial tryptophan codons, as it was not observed in other codons (for example, the mitochondrial phenylalanine codon) or in nuclear-encoded tryptophan codons ( Fig. 4c ). Data from biological replicates showed that this was reproducible ( Supplementary Fig. S3A ). qRT–PCR measurements indicated comparable expression levels of the mutated tRNA(Trp) 5556G>A and tRNA(Trp) wt in wt and tRNA(Trp) 5556G>A mutant mitochondria ( Fig. 4d , upper panel). Moreover, immune-precipitation analysis of mitochondrial ribosomes showed comparable enrichment levels ( Fig. 4d , lower panel). This indicates that the 5556G>A mutation in mitochondrial tRNA(Trp) does not lead to rapid degradation and does not affect loading into the ribosomes. However, despite the dramatic changes observed in the distribution pattern of mitochondrial RPFs, the TE was not affected in the tRNA(Trp) 5556G>A sample ( Fig. 4e ). Altogether, our observations indicate that the expression of tRNA(Trp) 5556G>A enforces relocation of mitochondrial ribosomes to tryptophan codons. 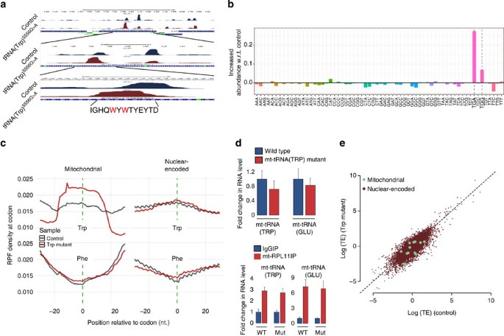Figure 4: tRNA(Trp)5556G>Acauses mitochondria malfunctioning and an increase of RPFs at tryptophan codons. (a) Screenshots from the UCSC genome browser showing RPFs of MT-CO2 gene in wt and tRNA(Trp)5556G>Amutant cybrids. (b) Differential codon abundance in the tRNA(Trp)5556G>Amutant cybrids compared with control wt. (c). The tRNA(Trp)5556G>Amutant cybrid (red line) shows increased RPF density with respect to wt controls (gray line) centered at tryptophan codon but not at a phenylalanine codons, nor at nuclear encoded codons (right panels). (d) Quantitative reverse transcriptase PCR (qRT–PCR) of tRNA(TRP) and control tRNA(GLU) from total RNA extracts from cybrids with either (Trp)5556G>Amutant or wt mitochondria (upper panel). Extracts from cybrids were immunoprecipitated by anti-mt-RPL11 or control IgG antibodies. Immunoprecipitated RNAs were detected by qRT–PCR using primers for mt-tRNA(TRP) and mt-tRNA(GLU) (lower panel). Mean values and s.d.’s were calculated from three independent experiments. (e) Log-transformed translational efficiencies in the (Trp)5556G>Amutant versus the wt control. Mitochondrially encoded genes are highlighted in green. Figure 4: tRNA(Trp) 5556G>A causes mitochondria malfunctioning and an increase of RPFs at tryptophan codons. ( a ) Screenshots from the UCSC genome browser showing RPFs of MT-CO2 gene in wt and tRNA(Trp) 5556G>A mutant cybrids. ( b ) Differential codon abundance in the tRNA(Trp) 5556G>A mutant cybrids compared with control wt. ( c ). The tRNA(Trp) 5556G>A mutant cybrid (red line) shows increased RPF density with respect to wt controls (gray line) centered at tryptophan codon but not at a phenylalanine codons, nor at nuclear encoded codons (right panels). ( d ) Quantitative reverse transcriptase PCR (qRT–PCR) of tRNA(TRP) and control tRNA(GLU) from total RNA extracts from cybrids with either (Trp) 5556G>A mutant or wt mitochondria (upper panel). Extracts from cybrids were immunoprecipitated by anti-mt-RPL11 or control IgG antibodies. Immunoprecipitated RNAs were detected by qRT–PCR using primers for mt-tRNA(TRP) and mt-tRNA(GLU) (lower panel). Mean values and s.d.’s were calculated from three independent experiments. ( e ) Log-transformed translational efficiencies in the (Trp) 5556G>A mutant versus the wt control. Mitochondrially encoded genes are highlighted in green. Full size image Next, we asked whether the relocation of ribosomes to tryptophan codons in the tRNA(Trp) 5556G>A mitochondria is a result of stalling, and therefore impacts on the downstream translation process. We aligned the first tryptophan of each mitochondrial transcript and plotted RPF density. Compared with wt mitochondria, tRNA(Trp) 5556G>A mitochondria manifested increased abundance of RPFs centered at the first tryptophan codons of mRNAs, and reduced abundance of RPFs downstream of it ( Fig. 5a ). This trait indicates stalling of the ribosome at tryptophan. To support global ribosome stalling, we aligned all mitochondrial transcripts and plotted RPF density along the transcripts. 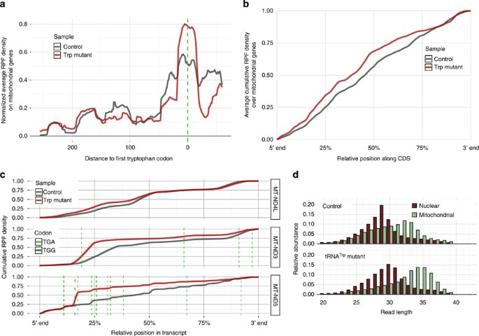Figure 5: tRNA(Trp)5556G>Astalls ribosomes at tryptophan codons and causes a change in RPF size distribution. (a) RPF density from the 5′ end of transcripts up to the first tryptophan codon occurrence averaged over the 13 protein-coding mitochondrial transcripts. (b) Cumulative RPF density normalized over the 13 protein-coding mitochondrial transcripts. (c) Example of the cumulative density of RPF density along the mitochondrial genes MT-ND4L (having no Trp codons), MT-ND3 and MT-ND5, in wt and tRNA(Trp)5556G>Amutant cybrids. (d) The relative abundance of RPF length in control and tRNA(Trp)5556G>Amutant cybrids. Figure 5b shows a cumulative density of RPFs and clearly indicates a significant reduction in RPF density at the 3′ half of the transcripts in the tRNA(Trp) 5556G>A mitochondria compared with tRNA(Trp) wt . Furthermore, this global effect was observed at the level of the individual transcripts. Figure 5c presents two examples (MT-ND3 and MT-ND5) of the change in RPF density along mitochondrial genes in tRNA(Trp) 5556G>A mutant and wt mitochondria. The change in RPF density generally showed good correlation with the appearance of tryptophan codons along the mitochondrial transcripts (green dashed lines in Fig. 5c and Supplementary Fig. S4 ), while the tryptophan-less MT-ND4L transcript showed a similar RPF pattern in control and mutant mitochondria. Thus, our results demonstrate the general effect of tRNA(Trp) 5556G>A mutation on mitochondrial translation, pausing ribosomes at tryptophan codons and altering ribosomal density on mitochondrial mRNAs. Figure 5: tRNA(Trp) 5556G>A stalls ribosomes at tryptophan codons and causes a change in RPF size distribution. ( a ) RPF density from the 5′ end of transcripts up to the first tryptophan codon occurrence averaged over the 13 protein-coding mitochondrial transcripts. ( b ) Cumulative RPF density normalized over the 13 protein-coding mitochondrial transcripts. ( c ) Example of the cumulative density of RPF density along the mitochondrial genes MT-ND4L (having no Trp codons), MT-ND3 and MT-ND5, in wt and tRNA(Trp) 5556G>A mutant cybrids. ( d ) The relative abundance of RPF length in control and tRNA(Trp) 5556G>A mutant cybrids. Full size image Last, the stalling of ribosomes in the tRNA(Trp) 5556G>A mutant mitochondria presented us with the possibility to examine the RPFs generated during ribosome progression. In particular, whether stalled ribosomes preferentially produce a certain type of RPFs. As tryptophan codons are enriched at the center of the RPFs in the tRNA(Trp) 5556G>A mutant mitochondria, our model ( Fig. 3d ) predicts accumulation of long RPFs. Figure 5d shows that ribosomes from cybrids with tRNA(Trp) 5556G>A mitochondria produce longer RPFs than cells with wt mitochondria. This phenomenon was reproduced in biological replicates ( Supplementary Fig. S3B ). A very moderate increase in cytosolic RPFs was observed too, perhaps due to metabolic changes the cells experience in the presence of dysfunctional mitochondria. Altogether, our results show, for the first time at a nucleotide resolution, how a mutation in tRNA disturbs translation, and how this information can be used to decipher ribosome progression. Impaired mitochondrial protein translation affects organismal development, function and ageing, and is a cause for early mortality in humans. Precise measurement of protein translation in the mitochondria is therefore crucial in understanding why malfunctioning occurs. Distinct characteristics of mitochondrial and cytosolic translation machineries however hampered faithful translation measurements using ribosomal profiling. By including several modifications to the ribosomal profiling protocol we show that efficient capturing of cytosolic and mitochondrial ribosomes RPFs in a single experiment is possible. Our adapted protocol provides a useful new tool for mitochondrial research. It allowed us to show that a genetic disorder caused by a mutated tRNA(Trp) 5556G>A leads to stalling of ribosomes on mitochondrial genes. The stalled positions are strongly enriched for tryptophan codons, and inversely tryptophan codons show a large increase in RPFs with respect to wt mitochondria. Furthermore, mitochondria expressing tRNA(Trp) 5556G>A showed an increase of ribosomes at the 5′ half of transcripts, and a decrease at the 3′ half. Thus, the point mutation in the mitochondrial-tRNA encoding for tryptophan has a vast effect on ribosome progression and rate of translation along the transcripts. We did not detect any prominent change in the translation in the cytosol, indicating limited effect to the mitochondria. Intriguingly, not all mitochondrial tryptophan codons induced stalling ( Fig. 5c and Supplementary Fig. S4 ), suggesting that other factors, such as mRNA structure, modification and composition, might influence the usage of mutated tRNA by mitochondrial ribosomes. Our findings also infer, for the first time, mitochondrial ribosome progression from sequencing-based data analyses. Mitochondrial ribosomes display a bi-modal size distribution of RPFs, peaking at 27 and 33 nt, in contrast to the single peak at 30 nt observed from cytosolic ribosomes. This observation suggests a parallel between mitochondrial and bacterial ribosomes, since a similar observation was recently made for the latter [13] . Altogether, the distribution of mitochondrial RPFs, their relative position with respect to mRNA, and changes due to a disease-causing tRNA mutation, suggest a model for ribosome movement ( Fig. 3d ) and stalling ( Fig. 6 ). 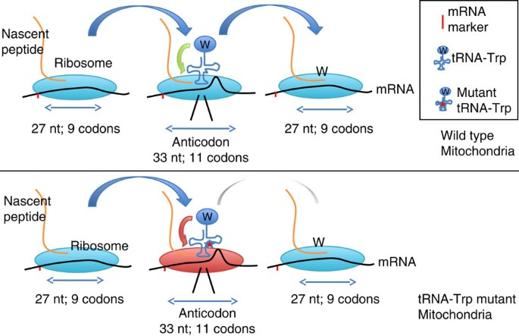Figure 6: Model for ribosome stalling. (a) Schematic model for ribosome stalling at codons translated by affected tRNAs, explaining the unbalanced generation of long RPFs in mutant mitochondria. Figure 6: Model for ribosome stalling. ( a ) Schematic model for ribosome stalling at codons translated by affected tRNAs, explaining the unbalanced generation of long RPFs in mutant mitochondria. Full size image RNA sequencing RNA was isolated using Trizol reagent (Invitrogen). RNASeq libraries were prepared using the TruSeq RNA Sample Prep Kit v2 (Illumina) following the manufacturer’s instructions. In brief, RNA was fragmented, then first-strand cDNA was prepared using the kit-supplied 1st Strand Master Mix and Superscript III (Life Technologies) followed by second strand cDNA synthesis. Libraries were amplified by PCR for 12 cycles and sequenced on a HiSeq 2000 System (Illumina). Alignment of raw data 5′ and 3′ adapters were clipped from ribosome profiling reads prior to alignment. rRNA and tRNA fragments were cleaned by aligning to databases of rRNA and tRNA (compiled from Ensembl ( http://dec2011.archive.ensembl.org/index.html ) categories ‘rRNA’, ‘rRNA_pseudogene’ and ‘Mt_rRNA’ and the genomic tRNA database [14] for hg19 respectively) in two alignment steps and removing reads with one or more hits. Cleaned data was aligned to hg19 using Tophat [15] and splice junctions of the transcriptome that was assembled by merging Ensembl, Refseq and Broad novel transcripts [16] using the gffread utility supplied with the cufflinks package [17] . Only primary alignments (that is, not having SAM flag 0x256) with mapping quality ≥10 were kept. Size distribution analysis Valid alignments were assigned to genes using htseq-count ( http://www-huber.embl.de/users/anders/HTSeq/doc/overview.html ) and only reads unambiguously assigned to a gene were counted. The gene-wise read density over the read sizes was averaged across genes with at least 100 reads. Periodicity analysis Coding sequence (CDS) regions were extracted from Ensembl and the 5′ ends of reads were offset 12 nucleotides in the 5′ direction to match the P-site location of ribosomes (that is, the currently ‘read’ codon). If reads aligned unambiguously to a single gene and unambiguously to a single frame of one or more transcripts of that gene they were assigned to that frame. TE analysis Genewise readcounts (in CDS for ribosome profiling data; over all exons for RNAseq data) were obtained using htseq-count (in ‘union’ mode, the default) and Ensembl annotations. Translational efficiencies were calculated as the normalized ratios (by total read counts) of RNAseq and ribosome profiling data over the mitochondrial genes. TMM normalization was applied to RNAseq and ribosome profiling data using the R package ‘edgeR’ [18] . Correlation of short and long RPFs Abundances of RPFs of 27 and 33 nt in length per mitochondrial protein coding transcript were used to calculate cross-correlation. The cross-correlation values were adjusted by multiplying with the length of the transcript. The normalized cross-correlation was averaged over the 13 transcripts. Codon enrichment RPFs assigned uniquely to the CDS of a mitochondrial gene were used to determine codon enrichment. For each RPF the current P-site was estimated by adjusting 17 nt from the 5′ end of the RPF. Only P-sites which were in-frame with the CDS were counted. The total number of each of the 64 codon occurences was counted in the control and mutant sample, and the relative frequencies were calculated. From this, the differences between mutant and control were calculated. Cell culture and western blotting BJ primary fibroblast and cybrid cells were cultured in DMEM supplemented with 10% heat-inactivated fetal calf serum (FCS) in 5% CO 2 at 37 °C. Cell extracts were separated on 10% SDS–PAGE gels and transferred to Immobilon-P membranes (Milipore). Antibodies used were mt-RPL11 (Cell Signaling, 1:1,000), RPL10a (Santa Cruz, 1:1,000), RPL7 (Abcam, 1:1,000) and RPS6 (Cell Signaling, 1:1,000). Validation and homoplasmy of the cybrids harboring the tRNA(Trp) 5556G>A mutation were verified by tRNA sequences obtained in the ribosome profiling protocol (see Supplementary Fig. S6 , which also shows full-length images of immunoblots). Ribosome profiling Approximately 30 × 10 6 cells were treated with chloramphenicol (100 μg ml −1 ) for 15 min and cycloheximide (100 μg ml −1 ) for 5 min. Cells were lysed in buffer B (20 mM Tris–HCl, pH 7.8, 100 mM KCl, 10 mM MgCl2, 1% Triton X-100, 2 mM DTT, 100 μg ml −1 chloramphenicol, 100 μg ml −1 cycloheximide, 1 × Complete protease inhibitor). Lysates were centrifuged at 1300 g and the supernatant was treated with 2 U μl −1 of RNase I (Ambion) for 40 min at room temperature. Lysates were fractionated on a linear sucrose gradient (7–47%) using the SW-41Ti rotor at 36,000 r.p.m. (221632.5 g ) for 2 h. Fractions enriched in mito-monosomes and cytosolic monosomes were identified by western blotting, pooled and treated with proteinase K (Roche) in 1% SDS. Released RPFs were purified using Trizol reagent (Invitrogen) following the manufacturer’s instructions. Libraries for deep sequencing were prepared as described previously [19] . In brief, digested fragments between 25–36 nucleotides were gel-purified and dephosphorylated using T4 polynucleotide kinase (New England Biolabs) for 5 h at 37 °C in buffer containing 100 mM MES-NaOH, pH 5.5, 10 mM MgCl 2 , 10 mM β-mercaptoethanol and 300 mM NaCl. 3′ adaptor was added with T4 RNA ligase 1 (New England Biolabs) for 2.5 h at 37 °C. Ligation products were 5′-phosphorylated with T4 polynucleotide kinase for 30 min at 37 °C. 5′ adaptor was added with T4 RNA ligase 1 for 2 h at 37 °C. All the sequencing experiments were performed on a HiSeq 2000 System (Illumina). Mitoribosome–tRNA complex inmunoprecipitation Cybrid cells were fixed with 1% formaldehyde for 10 min at 37 °C, quenched with 2.5 M glycine for 5 min and washed with 1 × PBS. Cell pellets were resuspended in lysis buffer (150 mM NaCl, 50 mM Tris, 0.5% Sodium deoxycholate, 0.2% SDS, 1% NP-40) supplemented with RNAseOUT (Invitrogen) and Complete protease inhibitors (Roche). Protein-G beads were washed and pre-incubated with mt-RPL11 antibody (Cell Signaling) (1:100) for 1 h at room temperature. Extracts and beads were incubated at 4 °C for 1 h. Beads were washed thrice with 1 × PBS, 0.1% SDS, 0.5% NP-40 and twice with 5 × PBS, 0.1% SDS, 0.5% NP-40. RNA was reverse crosslinked in the presence of proteinase K (Roche) at 65° for 3 h. RNA was purified using Trizol reagent (Invitrogen). Primer sequences mt-tRNA(TRP) forward: 5′-GAAATTTAGGTTAAATACAGACCAAGA-3′; mt-tRNA(TRP) reverse: 5′-GAAATTAAGTATTGCAACTTACTGAGG-3′; mt-tRNA(GLU) forward: 5′-ACAACGATGGTTTTTCATATCATT-3′; mt-tRNA(GLU) forward: 5′-TTCTCGCACGGACTACAACC-3′; Gapdh forward: 5′-ACCCAGAAGACTGTGGATGG-3′; Gapdh reverse: 5′-TCTAGACGGCAGGTCAGGTC-3′ Accession codes: Ribosome profiling data has been deposited in NCBI Gene Expression Omnibus under accession codes GSM1047584 and GSM1047585 (using the unmodified RP protocol) and GSE48933 (using the adapted RP protocol). The corresponding RNA sequencing data has been deposited in NCBI Gene Expression Omnibus under accession codes GSM1041191 and GSM1041192 (for the unmodified RP protocol) and GSE48933 (for the adapted RP protocol). How to cite this article: Rooijers, K. et al. Ribosome profiling reveals features of normal and disease-associated mitochondrial translation. Nat. Commun. 4:2886 doi: 10.1038/ncomms3886 (2013).